Discovery of seifertite in a shocked lunar meteorite Many craters and thick regoliths of the moon imply that it has experienced heavy meteorite bombardments. Although the existence of a high-pressure polymorph is a stark evidence for a dynamic event, few high-pressure polymorphs are found in a lunar sample. α-PbO 2 -type silica (seifertite) is an ultrahigh-pressure polymorph of silica, and is found only in a heavily shocked Martian meteorite. Here we show evidence for seifertite in a shocked lunar meteorite, Northwest Africa 4734. Cristobalite transforms to seifertite by high-pressure and -temperature condition induced by a dynamic event. Considering radio-isotopic ages determined previously, the dynamic event formed seifertite on the moon, accompanying the complete resetting of radio-isotopic ages, is ~2.7 Ga ago. Our finding allows us to infer that such intense planetary collisions occurred on the moon until at least ~2.7 Ga ago. The existence of a high-pressure polymorph in a meteorite suggests that its parent body has gone through a dynamic event [1] , [2] , [3] , [4] , [5] , [6] , [7] . Several previous studies have proposed that few high-pressure polymorphs are contained in lunar meteorites [8] , [9] although many craters and thick regoliths of the moon imply that it has experienced heavy meteorite bombardments. A recent study, however, revealed that a lunar meteorite, Asuka 881757, contains high-pressure polymorphs of silica, coesite and stishovite formed by meteorite bombardment 3.800 Ma ago [10] . Synthetic experiments indicate that silica transforms to coesite, stishovite, CaCl 2 -type, α-PbO 2 -type (seifertite) and pyrite-type forms as pressure and temperature rise [11] , [12] , [13] . There is still no clear evidence for the existence of post-stishovite phases in lunar meteorites. However, the occurrence and nature of high-pressure polymorphs of silica are still enigmatic in lunar meteorites. Notably, most silica grains in lunar meteorites and Apollo samples are cristobalite. The mechanism through which cristobalite transforms to its high-pressure polymorph has not been explained. These issues are not only important for understanding the dynamic events that have occurred on the Moon but they are also clues for exploring the Earth’s interior dynamics, because post-stishovite phases are expected to exist in the deep lower mantle and D″ layer in the core-mantle boundary of the Earth [12] , [14] . We investigated a lunar meteorite, Northwest Africa 4734 (hereafter, NWA 4734), and particularly a silica grain contained in the meteorite using a field-emission scanning electron microscope, an X-ray diffractometer (XRD), and a transmission electron microscope (TEM). NWA 4734 originated as lunar basalt. NWA 4734 showed many shock features such as shock veins and the presence of maskelynite, indicating that it was heavily shocked. We report robust evidence for the existence of seifertite, which was found only in a shocked Martian meteorite so far [15] , [16] , [17] , in a shocked lunar meteorite, NWA 4734, along with coesite and stishovite confirmed by X-ray and electron beam analyses. We also clarify the nature, occurrence and formation mechanism of seifertite. The identification of seifertite There are many silica grains in NWA 4734 that are about 100 μm in size, and they contain small amounts of Al 2 O 3 (0.59–0.99 wt%) and Na 2 O (0.21–0.26 wt%) ( Supplementary Table S1 ). Such impurities also exist in the silica of Martian and lunar meteorites [15] , [18] . Although most of silica grains in the shock veins are amorphous, some near the shock vein wall contain coesite ( Fig. 1a ). TEM images show that nano-size coesite crystal assemblages exist in the silica grains (Fig. 3a). We found many silica grains with a tweed-like texture ( Fig. 1c ), similar to silica grains in a Martian meteorite known as Shergotty, which contains seifertite [15] , [16] , [17] . Aoudjehane and Jambon [19] also observed similar silica grains in NWA 4734, and proposed that they might be seifertite based on their cathodoluminescence (CL) spectrum, although there is no standard spectrum to identify seifertite. Most of the tweed-like silica grains in NWA 4734 lie close to shock veins. Silica grains with a lamellae-like texture become dominant as the distance from the shock vein increases ( Fig. 1d ). Those grains have well-developed fractures, different from silica grains that have coesite in their shock veins and the tweed-like grains in and around the shock veins. Raman and CL spectroscopy revealed that some silica grains with lamellae-like textures contain stishovite. Blocks of the tweed-textured silica grains (~20 × 10 × 5 μm 3 ) were extracted by a focused ion beam (FIB) system and scanned with a synchrotron X-ray beam. The XRD patterns indicate that the silica grains consist of seifertite ( Fig. 2 ) with representative lattice parameters of a =4.078 (1) Å, b =5.030 (2) Å, c =4.483 (1) Å, V =91.96 Å 3 and space group=Pbcn ( Supplementary Table S2 ). The lattice parameters coincide with the seifertite contained in Shergotty [16] . In some cases, a small amount of stishovite accompanies seifertite. TEM images show that the seifertite crystals are rhomboid or spindle in shape and have dimensions of 50–200 nm by 100–600 nm ( Fig. 3b ). The dimensions of the seifertite crystals appear to become coarser near the shock vein. Each seifertite crystal is oriented parallel to its long axis. Seifertite crystals are surrounded with amorphous silica. 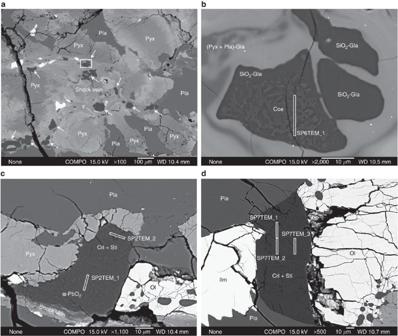Figure 1: Back-scattered electron images. (a) One shock vein intersects the other shock vein. White arrows indicate silica grains entrained in the crossed shock veins. (b) Magnified image of the boxed area in (a). (c) A silica grain adjacent to a shock vein. (d) A silica grain far from a shock vein. TEM slices prepared using a FIB are indicated by white boxes with numbers. Cri, cristobalite; Coe, coesite; Sti, stishovite; α-PbO2, seifertite; SiO2-Gla, silica glass; Ol, olivine; Pyx, pyroxene; Pla, plagioclase glass; Ilm, ilmenite. Figure 1: Back-scattered electron images. ( a ) One shock vein intersects the other shock vein. White arrows indicate silica grains entrained in the crossed shock veins. ( b ) Magnified image of the boxed area in ( a ). ( c ) A silica grain adjacent to a shock vein. ( d ) A silica grain far from a shock vein. TEM slices prepared using a FIB are indicated by white boxes with numbers. Cri, cristobalite; Coe, coesite; Sti, stishovite; α-PbO 2 , seifertite; SiO 2 -Gla, silica glass; Ol, olivine; Pyx, pyroxene; Pla, plagioclase glass; Ilm, ilmenite. 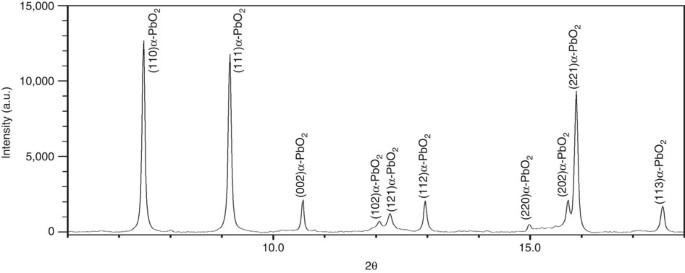Figure 2: Representative XRD patterns for seifertite. α-PbO2, seifertite. Full size image Figure 2: Representative XRD patterns for seifertite. α-PbO 2 , seifertite. 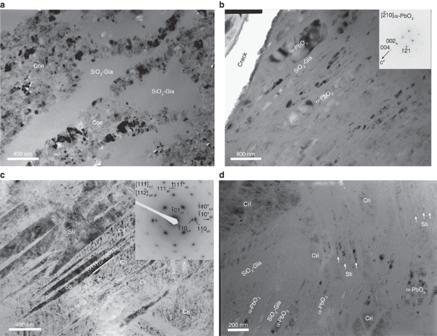Figure 3: TEM images. (a) Coesite in the silica grains entrained in shock veins (Fig. 1b) is assemblages of nano-size crystals. (b) Seifertite in the silica grain is rhomboid or spindle-shaped. Inserted selected area electron diffraction (SAED) patterns correspond to seifertite. (c) Thin stishovite platelets are stacked in cristobalite in the silica grains far from the shock vein. Inserted SAED patterns show {011}cri//{201}sti. (d) Seifertite and fragments consisting of cristobalite + stishovite coexist in intricate arrangements in the area between the seifertite-dominant and stishovite-dominant portions. Cri, cristobalite; Coe, coesite; Sti, stishovite; α-PbO2, seifertite; SiO2-Gla, silica glass. Full size image Figure 3: TEM images. ( a ) Coesite in the silica grains entrained in shock veins ( Fig. 1b ) is assemblages of nano-size crystals. ( b ) Seifertite in the silica grain is rhomboid or spindle-shaped. Inserted selected area electron diffraction (SAED) patterns correspond to seifertite. ( c ) Thin stishovite platelets are stacked in cristobalite in the silica grains far from the shock vein. Inserted SAED patterns show {011} cri //{201} sti . (d) Seifertite and fragments consisting of cristobalite + stishovite coexist in intricate arrangements in the area between the seifertite-dominant and stishovite-dominant portions. Cri, cristobalite; Coe, coesite; Sti, stishovite; α-PbO 2 , seifertite; SiO 2 -Gla, silica glass. Full size image Phase transition from cristobalite to stishovite or seifertite A synchrotron XRD and TEM observations show that the lamellae-like textured silica grains consist mainly of α-cristobalite ( a =5.063 (4) Å, c=6.99 (1) Å and space group=P4 1 2 1 2) ( Supplementary Table S3 ). Some cristobalite (cri) crystals have a twin structure with a twin plane {110} cri . Stishovite ( a =4.204 (3) Å, c =2.678 (5) Å and space group=P42/mnm) ( Supplementary Table S4 ) platelets with a thickness of 50–200 nm are stacked in the twinned cristobalite ( Fig. 3c ). We found a specific crystallographic orientation between the twinned cristobalite and stishovite (sti) platelets; {011} cri //{201} sti . In some cases, amorphous silica exists between the cristobalite and stishovite platelets. Seifertite and fragments including cristobalite + stishovite platelets coexist in the area between tweed-like silica grains and lamellae-like silica grains ( Fig. 3d ). We could not identify a specific crystallographic orientation of the seifertite and fragments including cristobalite + stishovite platelets. Detailed chemical compositions and lattice parameters of cristobalite, stishovite and seifertite are in the Supplementary Information . Representative Raman and CL-spectrum data are also included in the Supplementary Information ( Supplementary Figs S1,S2 ). High-temperature (β-) cristobalite (cubic) transforms easily to low-temperature (α-) cristobalite (tetragonal) around 500 K (ref. 20 ). Most of the cristobalite in NWA 4734 is α-cristobalite. Most of it in the Apollo samples has twinning and curved fractures, indicating that it inverted from β-cristobalite to α-cristobalite during cooling [20] , [21] . When β-cristobalite transforms back to α-cristobalite, stacking faults are induced along {011} of the α-cristobalite, equivalent to {111} of β-cristobalite [22] . It is likely that nucleation takes place along the stacking faults in the high-pressure and -temperature conditions induced by dynamic events. Subsequently, stishovite platelets grow. The lamellae-like silica grains are similar to quartz grains with stishovite lamellae in lithic clasts of the Ries impact crater [23] . The transformations from quartz to stishovite and from cristobalite to stishovite would both be activated by coherent phase transition mechanism because topotaxial relationships exist between them. The pressure-temperature phase diagram deduced from synthetic experiments using cristobalite as a starting material shows that stishovite or seifertite appears at pressure conditions between ~50 and ~90 GPa, and temperature conditions between ~500 and ~2,500 K ( Fig. 4 ) (refs 24 , 25 ). Seifertite appears instead of stishovite at similar pressures, but higher temperatures. This coincides with the transformation from cristobalite to stishovite or seifertite observed in the shock veins of NWA 4734. TEM observations show that cristobalite had transformed to seifertite near the shock veins, whereas cristobalite had transformed to stishovite farther from them; that is, cristobalite transformed to seifertite in hotter portions, but to stishovite in colder portions under the same pressure. These occurrences imply that the Clapeyron slope between stishovite and seifertite is negative, even though there is some disagreement, based on deductions from synthetic experiments, about the Clapeyron slope between stishovite and seifertite (or CaCl 2 -type silica) [12] , [25] , [26] . Cristobalite becomes unstable as pressure and temperature increase in a dynamic event. Nucleation takes place around the cristobalite fragments, and seifertite grows. The grains of the seifertite crystals are coarser near the shock veins than they are farther away, implying that the grain growth of seifertite crystals depends on temperature. Most seifertite is accompanied by amorphous silica. Although we cannot rule out the possibility that the amorphous silica originates from other high-pressure polymorphs of silica [27] , it is likely that seifertite became amorphous partly by residual heat during a decompression stage. The pressure at which coesite is stable is lower than that of stishovite and seifertite. Although abundant seifertite might also have existed in the silica grains entrained in the shock veins, it would have been vitrified during the decompression stage. Finally, rapid-growth of coesite might have occurred in the vitrified silica. 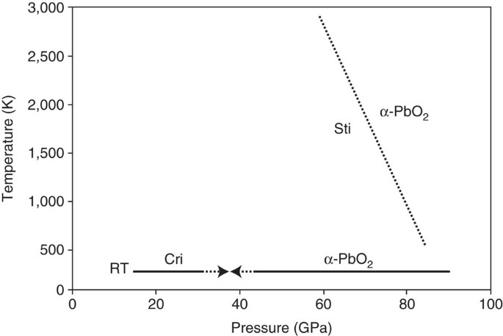Figure 4: Pressure-temperature phase diagram. Dubrovinskyet al.25is modified. Cri, cristobalite; Sti, stishovite; α-PbO2, seifertite; RT, room temperature. Figure 4: Pressure-temperature phase diagram. Dubrovinsky et al . [25] is modified. Cri, cristobalite; Sti, stishovite; α-PbO 2 , seifertite; RT, room temperature. Full size image We could estimate the pressure condition recoded in NWA 4734 based on high-pressure polymorphs of silica. The pressure–temperature phase diagram shows that cristobalite transforms to seifertite at ~40 GPa under room temperature condition ( Fig. 4 ). However, we cannot adopt it for NWA 4734 because the shock vein including seifertite shows clear evidence for melting. Cristobalite transforms to seifertite above about 60 GPa at around 2,500 K (ref. 25 ) ( Fig. 4 ). The phase diagram was obtained by synthetic experiments using pure cristobalite as a starting material. The cristobalite in NWA 4734, however, contains a small amount of aluminium and sodium. Some previous works indicate that, for alumina-bearing silica, the phase boundary between stishovite and CaCl 2 -type silica shifts considerably to a lower pressure condition [28] , [29] . The effect of sodium on the phase boundary has not yet been evaluated. Although the phase boundary between stishovite and seifertite using alumina- or sodium-bearing cristobalite as a starting material has not been determined, it is likely that the phase boundary also shifts to a somewhat lower pressure condition. Nonetheless, the pressure condition recoded in NWA 4734 would be ~40 GPa or more. The melting temperature of NWA 4734 would be similar to those of KLB-1 peridotite and Allende meteorite [30] , [31] , [32] . Expected temperature in the shock vein would be 2573 K or more (corresponding to the liquidus temperature of KLB-1 peridotite and Allende meteorite). The 40 Ar- 39 Ar radio-isotopic age of NWA 4734 obtained from bulk-fragment, pyroxene and feldspar is ~2.7 Ga [33] , which is a little younger than its 207 Pb- 206 Pb radio-isotopic age (~3073 Ma) [18] . 40 Ar- 39 Ar radio-isotopic age is sensitive to temperature. Several previous studies show evidences that a dynamic event can modify 40 Ar- 39 Ar radio-isotopic ages [34] , [35] , [36] , [37] , [38] . 40 Ar- 39 Ar radio-isotopic spectrum of NWA 4734 shows a broad ‘plateau’ at ~2.7 Ga [33] , implying that the 40 Ar- 39 Ar system was completely reset. Recent studies quantified minimum time required for complete resetting of 40 Ar- 39 Ar system using argon diffusion coefficient [37] , [39] . Temperature history recorded in NWA 4734 is an important factor for calculation. A high-pressure polymorph vitrifies easily by heat at atmospheric pressure condition. For instance, silicate-perovskite [(MgFe)SiO 3 ] instantaneously vitrifies by heat of 150 °C at atmospheric pressure condition [40] . Seifertite immediately vitrifies even by very weak Ar + laser (generating less heat) irradiation for Raman analysis or by electron beam irradiation during TEM observation. Seifertite can never survive a heat event inducing complete resetting of 40 Ar- 39 Ar system. Namely, seifertite formation age is never older than ~2.7 Ga. Feldspar (now maskelynite) is a major carrier for argon gas. Most of the maskelynite in NWA 4734 has smooth surfaces without fractures or planar defects. Feldspar was heated and subsequently melted, finally became amorphous by quenching during a dynamic event [38] , thus leading to degassing of argon. The bulk modulus of feldspar is smaller than those of olivine and pyroxene, for example, Matsui [41] . The melting temperature of feldspar is lower than those of olivine and pyroxene at same pressure condition. When the difference of bulk modulus between feldspar and surrounding minerals becomes extreme with increasing pressure condition induced by a dynamic event, stress concentrates on feldspar, thus leading to be heated locally beyond melting temperature (~2,000 K), for example, Birch and LeComte [42] . The duration of high-temperature during a dynamic event is also important factor for calculating the minimum time required for complete resetting of 40 Ar- 39 Ar system, and it is related with the duration of high-pressure condition. The formation of a high-pressure polymorph is kinetically controlled, for example, refs 43 , 44 , 45 . If the duration of high-pressure condition is too short, a high-pressure polymorph cannot form even if a shock vein is formed. Several previous studies estimated the duration of high-pressure condition in shocked meteorites including high-pressure polymorphs in and around shock veins using the kinetics of high-pressure polymorphs, for example, refs 3 , 4 , 46 . According to these previous studies, the duration of high-pressure condition is from mili second to several seconds. We need the growth rate of seifertite to estimate the duration of high-pressure condition recorded in NWA 4734. However, the kinetics data of seifertite have not been obtained so far. Seifertite and stishovite formed from cristobalite simultaneously during the dynamic event. The growth rate of stishovite from cristobalite also has not been studied. Nonetheless, we could use the grain growth rate of stishovite in MORB composition [47] for approximate estimation. The estimation was conducted by integrating the grain growth rate and thermal history. The estimated duration of high-pressure condition required for stishovite formation in NWA 4734 is ~0.1 s at least (details of calculation process are described in the Supplementary Information ). In addition, temperature decreases through thermal conduction is sluggish compared with pressure release. In conclusion, the young 40 Ar- 39 Ar radio-isotopic ages (relative to the 207 Pb- 206 Pb radio-isotopic ages) would be closely related with a dynamic event formed seifertite. Cosmic-ray exposure age of NWA 4734 is ~570 Ma [33] . There is no clear evidence for other dynamic events besides the dynamic event that formed the seifertite. Assuming that NWA 4734 was launched from the moon at ~570 Ma, the dynamic event was very weak and did not cause the increasing of pressure and temperature, otherwise seifertite and stishovite would vitrify. We could estimate the approximate size of asteroid collided on the moon using the estimated duration of high-pressure condition (>~0.1 s). The estimated size of asteroid collided on the moon is ~0.4 km at least, which formed a crater with a diameter of ~7 km at least (Details of calculation process are described in the Supplementary Information ). The latest surface observations show that the cumulative frequency of craters with a diameter of ~7 km or greater is ~10 −5 /km −2 around 2–3 Ga (Eratosthenian system) [48] . The area of mare basalt on the moon is ~7 × 10 6 km 2 (ref. 49 ). Assuming that the very approximate area of Eratosthenian system is ~50% of the mare basalt, the number of a crater having a diameter of ~7 km or greater is ~35. Although craters with a diameter of ~7 km are not so large among lunar craters, it is a relatively large among craters formed around 2–3 Ga. In addition, the estimated magnitude of the shock event is a lower limit, and would be considerably underestimated, because the growth rate of stishovite used here might be too fast. Coherent phase transition mechanism worked for the transformation from cristobalite to stishovite in NWA 4734. It is likely that there are significant differences on growth rates between coherent and incoherent phase transition mechanisms. For instance, in case of transformation from olivine to its high-pressure polymorph, ringwoodite, incoherent growth rate are two or three orders of magnitude faster than coherent growth rate [44] . The magnitude of the shock event formed seifertite and stishovite may be several orders of magnitude greater than the magnitude estimated here because we used the incoherent grain growth rate of stishovite in MORB composition [47] for approximate estimation (See the Supplementary Information ). A lunar meteorite, Northwest Africa 4881 (NWA 4881) shows a similar young 40 Ar- 39 Ar radio-isotopic age (~2.6 Ga) as NWA 4734 (ref. 50 ). The 40 Ar- 39 Ar radio-isotopic age of NWA 4734 and NWA 4881 is one of the youngest ages in chronology of the lunar meteorite clan. In other words, it is likely that such planetesimal collisions that induced complete resetting of 40 Ar- 39 Ar system (and formed high-pressure polymorphs) would be still occurring 2.7 Ga ago at least on the Moon. The 40 Ar- 39 Ar radio-isotopic age distribution of impact melts in lunar meteorites [51] would also support that such planetary collisions have continued till around 2.7 Ga on the Moon even after the late heavy bombardments (LHB: 3.8–4.1 Ga) period although it would not be so frequent like the LHB period, which would coincide with crater chronology [48] . Thus, the present results confirmed and strengthened the crater chronological view of the magnitude of collisions in 2–3 Ga on the moon based on the real materials, mineral physics and 40 Ar- 39 Ar radio-isotopic chronology. Oxygen increased on the Earth around 2.7 Ga ago because cyanobacteria erupted in the sea [52] , [53] . The Earth might have also still been suffering from such planetesimal collisions at that time because the Earth was much closer to the Moon [54] . The planetesimal collision might have destroyed developing biosphere on the Earth. One of the oldest craters on the Earth, the Vredefort dome in South Africa, is speculated to be 2.0 Ga old [55] . The Vredefort dome is one of the biggest craters on the Earth, implying that a mega-impact occurred 2.0 Ga ago. Recently, an evidence for older crater (3.0 Ga) was found in West Greenland [56] . However, most evidences for old impact events on the Earth would have been lost due to weathering and plate movement. Recent studies report high-pressure polymorphs of olivine, wadsleyite and ringwoodite together with those of silica in lunar meteorites [10] , [57] , [58] . These high-pressure polymorphs in lunar meteorites, overlooked over the years, might be a new clue for understanding the meteorite bombardments that has occurred on the early Moon and Earth. Petrologic description A polished NWA 4734 chip sample was prepared for this study. Its mineralogy was determined using a Laser micro-Raman, JASCO NRS-2000 spectrometer with a liquid nitrogen-cooled CCD detector. A microscope was used to focus the excitation laser beam. We also measured the CL spectrum to identify minerals using a scanning electron microscopy-CL apparatus comprising a SEM (JEOL: JSM-5410) combined with a grating monochromator (Oxford: Mono CL2) (accelerating voltage=15 kV and beam current=1.0 nA) equipped with a Gatan Mini-CL. Sensitivity calibration was conducted to reduce sensitivity dependence between the devices. We used a field-emission scanning electron microscope, JEOL JSM-71010 for detailed fine textural observations. An accelerating voltage of 15 kV was employed. Chemical compositions were determined using the wavelength-dispersive procedure of the JEOL JXA-8800M electron micro-probe analyser. Analyses were carried out using an accelerating voltage of 15 kV, a beam current of 10 nA and a defocused beam of 1–10 μm. Synchrotron XRD and TEM observation A part of the sample was excavated with a FIB system, JEOL JEM-9320FIB, and the extracted slice was placed on a culet of single diamond. The excavated samples on the diamond were scanned at the BL10XU beam line (SPring-8). A monochromatic incident X-ray beam with a wavelength of 0.41456(5) or 0.41297(7) Å was collimated to a diameter of <10 μm. XRD spectra were collected on an imaging plate using an exposure time of 5–30 min. The XRD spectrum of cerium dioxide (CeO 2 ) was used to determine the wavelength and the distance between the sample and the imaging plate. Slices for TEM observations were prepared using an FIB system. A JEOL JEM-2010 microscope operating at 200 kV was employed for conventional TEM observations and selected area electron diffraction. How to cite this article: Miyahara, M. et al . Discovery of seifertite in a shocked lunar meteorite. Nat. Commun. 4:1737 doi: 10.1038/ncomms2733 (2013).